Self-assembled ultrathin nanotubes on diamond (100) surface Surfaces of semiconductors are crucially important for electronics, especially when the devices are reduced to the nanoscale. However, surface structures are often elusive, impeding greatly the engineering of devices. Here we develop an efficient method that can automatically explore the surface structures using structure swarm intelligence. Its application to a simple diamond (100) surface reveals an unexpected surface reconstruction featuring self-assembled carbon nanotubes arrays. Such a surface is energetically competitive with the known dimer structure under normal conditions, but it becomes more favourable under a small compressive strain or at high temperatures. The intriguing covalent bonding between neighbouring tubes creates a unique feature of carrier kinetics (that is, one dimensionality of hole states, while two dimensionality of electron states) that could lead to novel design of superior electronics. Our findings highlight that the surface plays vital roles in the fabrication of nanodevices by being a functional part of them. The outstanding mechanical, thermal, optical and electronic properties of carbon nanotubes (CNTs), the largest family of sp 2 carbon materials, have been intensively investigated for various applications [1] , [2] , [3] since the discovery of CNTs in 1991 (ref. 4 ). Recently developed ultrathin CNTs with diameters as small as a few angstroms [5] , [6] show distinct electronic properties that arise from their tight curvature bending on the sp 2 orbitals [7] , [8] . However, the great curvature limits their formation, and the smallest tubes synthesized have been formed only inside other nanotubes. Unlike CNTs, bulk diamond consists of sp 3 hybridized C. However, the hybridization of C at an abrupt and unpassivated surface should be fundamentally different from that in the bulk. The otherwise dangling bonds (DBs) of sp 3 C on a diamond surface are usually eliminated via reconstructions that involve the formation of new bonds. Of the low-index diamond surfaces, only the (100) surface has two DBs per terminated surface C (the (110) or the (111) surface has only one). The (100) surface is the dominant surface in ultrananocrystalline diamond and in diamond thin films formed by chemical vapour deposition [9] , [10] , [11] . A simple (2 × 1) reconstruction of this surface featuring a C=C dimer was proposed theoretically in 1981 (ref. 9 ) and observed in 2001 (ref. 11 ). No other surface reconstruction with competing structural stability has yet been proposed. The determination of a material’s surface structure is an important but challenging step towards understanding its effects on the performance of devices [12] . Experimental studies are often impeded by the complicated surface reconstructions that semiconductors undergo. Observation is also severely disturbed by chemical processes such as surface oxidation. On the theory side, numerous surface reconstruction simulations have been carried out, most of which rely on educated guesses for structures either known from other materials or initialized by chemical intuition (for example, ref. 10 ). Only a few automatic surface structure-searching methods based on basin hopping [13] and genetic algorithms [14] , [15] were previously attempted, and the results showed an advantage of these searching algorithms. There is a growing need on the intelligent structure-searching method for surface characterization that does not rely on any prior known surface structure information. Here we present an automatic surface structure-searching method that employs structure swarm intelligence, a technique recently developed for finding the global minimum in a complex configuration space [16] , [17] . Search efficiency is improved by implementing symmetry groups and by applying chemical constraints on the surface structures. The application of our method to analyse the structure reconstructions of the diamond (100) surface unexpectedly reveals a spontaneous formation of arrays of self-assembled CNTs. The formation energy of such a surface reconstruction is competitive with that of the known dimer surface structure. Under certain external conditions (a small compressive strain or a high temperature), the self-assembled CNTs surface becomes the more stable reconstruction structure. Surface reconstruction searching method The swarm intelligence algorithm via particle-swarm optimization represents the motions and evolutions of natural populations such as flocking birds or schooling fish [18] . It has been widely used to explore the global minima of many other nonlinear systems with complicated configuration spaces. Swarm intelligence has recently been introduced into the CALYPSO algorithm [17] for the structure searching of extended crystals, layered materials and nanoparticles [16] , [17] , [19] , [20] , resulting in the successful prediction of the crystal structures of many compounds [21] . Our approach is outlined in Fig. 1a . An ensemble of surface structures is initially constructed unbiasedly by depositing a fixed number of atoms on an ideal surface. The atoms are randomly attached to the surface with bonds to at least one original surface atom. Symmetry operations of various two-dimensional space groups are applied while constructing the initial surface structures. Surfaces of semiconductors with a sizable band gap, such as diamond, are also handled using the electron-counting rules (ECR) [22] , [23] , which generally require bonding states and anion DB states to be filled with electrons, while anti-bonding and cation dangling bonding states are required to be vacant. Symmetry operations resulted in a greatly reduced search space. ECR enabled efficient surface structure searching. 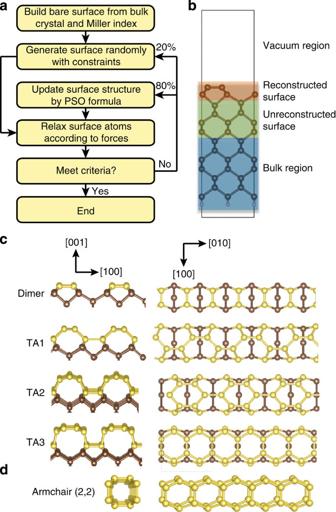Figure 1: Surface structure-searching scheme and predicted surface structures. (a) The programme chart of CALYPSO module for searching surface structures. (b) A sketch of the slab model. It typically consists of three regions: the bulk region, the unreconstructed surface and the reconstructed surface. The bulk region contains 6–8 layers. The bottom side of the slabs is passivated by hydrogen atoms with integer or partial charges. The atoms in the bulk region of the slab model are fixed so as to reserve the bulk nature of the materials. The atoms in the unreconstructed surface region (2–4 layers) are relaxable but not to be involved in the structure evolution. The atoms in the reconstructed surface region are subject to structure swarm evolution. Note that in practice, the reconstructed surface region is not limited to two layers, and can be more layers dependent on the energetic situation of systems. (c) The predicted surface structures at the diamond (100) surface. Left and right panels are side and top views, respectively. (d) Armchair (2, 2) CNTs was plotted for comparison. Figure 1: Surface structure-searching scheme and predicted surface structures. ( a ) The programme chart of CALYPSO module for searching surface structures. ( b ) A sketch of the slab model. It typically consists of three regions: the bulk region, the unreconstructed surface and the reconstructed surface. The bulk region contains 6–8 layers. The bottom side of the slabs is passivated by hydrogen atoms with integer or partial charges. The atoms in the bulk region of the slab model are fixed so as to reserve the bulk nature of the materials. The atoms in the unreconstructed surface region (2–4 layers) are relaxable but not to be involved in the structure evolution. The atoms in the reconstructed surface region are subject to structure swarm evolution. Note that in practice, the reconstructed surface region is not limited to two layers, and can be more layers dependent on the energetic situation of systems. ( c ) The predicted surface structures at the diamond (100) surface. Left and right panels are side and top views, respectively. ( d ) Armchair (2, 2) CNTs was plotted for comparison. Full size image Once the initial structures are generated, their geometries are optimized using first principles density functional theory (DFT); their total energies are also calculated. The structures then evolve towards lower-energy structures, locally and globally, through self- and swarm-structure learning. To enhance structural diversity and to ensure unbiased structure generation and the coverage of the entire configuration space, a changeable amount of random structures (typically 20%) is created and included in each structure generation calculation. Our method has been incorporated into CALYPSO code [17] and successfully benchmarked against the known surface reconstructions of various semiconductors, including C, Si, SiC, AlN, and ZnO. Experimentally observed surfaces are readily reproduced by the surface structure-searching method from input knowledge of only the chemical compositions. Self-assembled CNTs on diamond (100) surface The developed method successfully reproduces the experimentally observed dimer structure on a diamond (100) surface, but several other energetically comparable, low-energy structures are also identified ( Supplementary Fig. 1 ). Some appear to be variations of the dimer structure, but other, unexpected and previously unknown surface reconstructions contain self-assembled CNT arrays (structures labelled TA1, TA2 and TA3 in Fig. 1c ). These structures consist of a large number of sp 2 hybridized C atoms, which can be considered as arrays of radially deformed single-walled CNTs on the diamond (100) surface. The tube arrays possess five-, seven- and eight-membered C rings, with the bottom of each being embedded on the diamond (100) surface. The static energy of TA1, calculated using DFT within the Perdew–Burke–Ernzerhof (PBE) functional [24] at 0 K, is greater than that of the dimer by only 3.8 meV per (1 × 1) unit cell. The other arrays, TA2 and TA3, are less favourable than TA1 by 0.421 and 0.162 eV per (1 × 1) unit cell, respectively. Given the extremely small energy difference between TA1 and the dimer, various other functionals are also tested to compare the structures’ relative stability ( Supplementary Table 1 ). Both structures are consistently found to be energetically competitive at 0 K. Note that while surface supported CNTs have been previously studied by both first-principle calculations and experiment [25] , [26] , such studies have typically examined nanotubes bound on the surface by van der Waals forces or weak chemical bonds, in fundamental contrast to the self-assembled, chemically bonded tube arrays of the present work. The C atoms in the top two layers (gold colour in Fig. 1c ) of the TA1 structure each form bonds with three other C atoms, topologically similar to those in conventional nanotubes. The distances between nearest and next-nearest neighbouring C atoms are 1.453 and 1.539 Å, featuring double C=C and single C–C bonds, respectively, and they are distributed alternately along the tube direction. Differences arise in the lower half of each tube, where each C atom bonds with four others. Note that the C=C bond length of the TA1 structure is much longer than the 1.382 Å in the dimer structure. This elongation is the result of the small radius of the tube: geometric constraints lead to excessively bent sp 2 hybridization. Tube radius increases in the series of arrays from TA1 to TA3, with a single tube in TA3 resembling an isolated (2,2) CNT [27] ( Fig. 1d ), the smallest nanotube yet observed. Surface structure stability The energetic stabilities of the self-assembled CNT structures can be considerably enhanced by external perturbations, such as compressive strain or heating ( Fig. 2a,b ). The structural stabilities of TA1 and the dimer structure are compared under three typical compressive strains (uniaxial (100) and (010), and biaxial) ( Fig. 2a ). Uniaxial (100) strain induces the energy of the TA1 structure to decrease and that of the dimer structure to increase; a very small strain of 0.12% is sufficient to reduce the static energy of TA1 at 0 K to below that of the dimer structure. Compressive (010) strain reduces the energies of both structures, but more in TA1, allowing it to prevail over the dimer at a strain of 0.18%. Similarly, a biaxial compressive strain of 0.12% leads TA1 to be more stable than the dimer. Note that the use of the Heyd–Scuseria–Ernzerhof (HSE) functional [28] further supports the results obtained using the PBE functional ( Fig. 2a ). Small strains of less than 0.2% can be readily applied on a diamond surface through its growth on different substrates. High-temperature growth can lead to large in-plane compressive strains in diamond films upon their cooling once formed [29] . 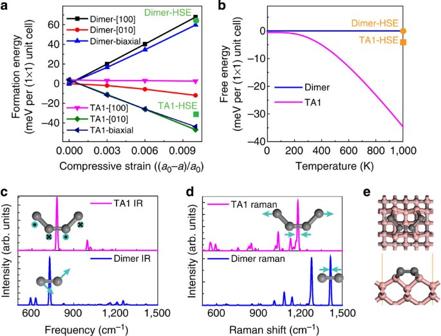Figure 2: External influences on the stability of dimer and TA1 structures, and simulated spectra. (a) The static surface energies within PBE functional as a function of strains applied along (100) and (010), and biaxially. Compressive strain is represented by the relative lattice compression ratio, that is, (a0−a)/a0, in whichaanda0are the compressed and balance lattice parameter respectively. Results (large symbols marked by green) derived from HSE functional at 1% biaxial compressive strain was shown for comparison. (b) The relative surface Gibbs free energies within PBE functional of TA1 structure with respect to dimer structure as a function of temperature. The data (symbols) derived from HSE functional at 1,000 K was also shown for comparison. (c,d) The calculated IR and Raman spectra of TA1 and dimer surface structures. The structural motifs seen in the insets are depicted inefor TA1 and dimer structures, respectively. Figure 2: External influences on the stability of dimer and TA1 structures, and simulated spectra. ( a ) The static surface energies within PBE functional as a function of strains applied along (100) and (010), and biaxially. Compressive strain is represented by the relative lattice compression ratio, that is, ( a 0 − a )/ a 0 , in which a and a 0 are the compressed and balance lattice parameter respectively. Results (large symbols marked by green) derived from HSE functional at 1% biaxial compressive strain was shown for comparison. ( b ) The relative surface Gibbs free energies within PBE functional of TA1 structure with respect to dimer structure as a function of temperature. The data (symbols) derived from HSE functional at 1,000 K was also shown for comparison. ( c , d ) The calculated IR and Raman spectra of TA1 and dimer surface structures. The structural motifs seen in the insets are depicted in e for TA1 and dimer structures, respectively. Full size image The effects of temperature on the stability of the various surface structures are demonstrated in their phonon spectra calculated using the supercell method ( Supplementary Fig. 2 ). The dimer and all the self-assembled CNT structures are dynamically stable without having any imaginary phonon modes. Compared with the dimer structure, TA1 shows very different active infrared (IR) and Raman spectra ( Fig. 2c,d ). The IR spectrum exhibits distinguishing lines at 778 cm −1 and 996 cm −1 ; the former, the strongest signal, corresponds to C–C=C–C out-of-plane vibrations. These IR and Raman features can be used to identify the formation of the tube arrays on the diamond (100) surface. The Gibbs free energies of the dimer and TA1 are calculated within a quasi-harmonic approximation with respect to temperature up to 1,000 K ( Fig. 2b ). The inclusion of vibrational contributions in the energy calculations has multiple effects. First, within the PBE functional, the consideration of zero-point energy favours the self-assembled CNTs, as expected given the much stronger C=C bonding in the dimer than in the self-assembled CNTs. However, consideration of zero-point energy also leads the lattice to expand by ~0.35% ( Supplementary Fig. 3 ), increasing the energy of the self-assembled CNTs. The net result is that TA1 is energetically favoured over the dimer at 0 K, although the energy difference (0.57 meV per (1 × 1) unit cell) is within the error bar of our calculations. In contrast to the unresolvable energy order at 0 K, the Gibbs free energy calculated including temperature effects clearly shows the stabilization of the TA1 structure at elevated temperatures ( Fig. 2b ). Our PBE calculations reveal a large energy gain of TA1, reaching 35 meV per (1 × 1) unit cell at 1,000 K. Among the various functionals, HSE most greatly favours the dimer structure ( Supplementary Table 1 ); its use narrows the Gibbs free energy difference to 3.0 meV at 1,000 K (symbols in Fig. 2b ), while still indicating the greater energetic stability of TA1 at high temperature. Electronic structures The band structures and density of states (DOS) for TA1 illustrate its electronic properties ( Fig. 3a ). The structure is a semiconductor featuring a direct band gap at the zone boundary X point calculated to be 0.33 eV by the PBE functional and 0.96 eV by the HSE hybrid functional. The latter functional has been demonstrated to be more reliable for band gap calculations. Further calculations using GW [30] method found a band gap of 1.01 eV, which is quite close to the HSE result. 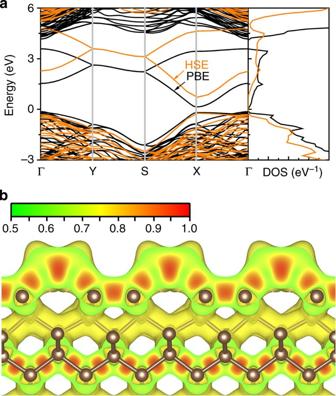Figure 3: Electronic structures and charge localization of TA1 surface. (a) The band structure and electronic DOS of TA1 surface. Black and brown lines are the band structure data obtained from the uses of PBE and HSE functionals, respectively; (b) The calculated ELF of TA1 surface. Green to red indicates the gradually increased charge localization. Figure 3: Electronic structures and charge localization of TA1 surface. ( a ) The band structure and electronic DOS of TA1 surface. Black and brown lines are the band structure data obtained from the uses of PBE and HSE functionals, respectively; ( b ) The calculated ELF of TA1 surface. Green to red indicates the gradually increased charge localization. Full size image There is a unique band structure feature around the X point ( Fig. 3a ). The lowest conduction band has a large dispersion in both X-S (axial to the tube) and X-Γ (radial to the tube) directions, whereas the highest valence band has a large dispersion only in the X-S direction and is quite flat in the X-Γ direction. The band structure indicates that the electrons can transport equally well axial and radial to the tubes. In contrast, hole transport is much easier along the tubes than across them, showing anisotropic or one dimensional transport behaviour. Therefore, the dimensionality of the carrier transportation on this self-assembled CNT surface is controllable by changing the carrier types (from electrons to holes), which can be achieved through doping or under an applied gate voltage. Chemical bondings The novel electronic properties of the self-assembled CNTs at the diamond (100) surface originate from their unique bonding features. The nature of their bonding was probed by calculating the electron localization functions (ELF) of TA1 ( Fig. 3b ). The C atoms on the top layer are sp 2 hybridized and form both σ and π bonds with their neighbouring C atoms. A basin of electron localization was found between the C atoms in neighbouring tubes, indicating the formation of covalent bonds between tubes. This bonding is quite unusual given that the C–C distance (1.788 Å) is notably longer than the longest reported C–C σ bond (1.704 Å) [31] . The formation of such a long C–C σ bond is actually not enforced by the proximity of the self-assembled tubes on the surface. A relaxation calculation was conducted for free tube arrays having the C atoms at the lower part of the tube passivated with hydrogen atoms, which was constructed by the removal of unreconstructed surface and the bulk regions out of simulation cell ( Supplementary Fig. 4 ). The optimized C–C distances between the tubes remained nearly invariant, and the covalent bonding persisted. Therefore, this unusually long C–C covalent bonding is intrinsic and closely related to the severely bending of the C atoms on the small tubes and the large deviation from ideal sp 2 behaviour. This distinctive feature weakens the C–C π bonding on the tube, but promotes covalent bondings between neighbouring tubes. The very different bonding topologies between the self-assembled CNTs and the dimer surface might lead to a large kinetic barrier that naturally suppresses the transition between them. A plausible transition path from TA1 to the dimer structure is proposed ( Supplementary Fig. 5 ); its fairly large activation barrier is calculated to be 1.59 eV per (1 × 1) unit cell using the nudged elastic band method [32] Such a large barrier would effectively prevent the transition. Therefore, a surface with tube arrays would likely be stable if used in electronic devices. Experimental scanning tunnelling microscopy measurements [11] have been performed to resolve the structure of diamond (100) surface, and the obtained array-like image has been attributed to the convolution of the wave functions of a dimer structure. However, the particular surface was prepared under hydrogen-rich conditions, which are preferable for the growth of the dimer structure ( Supplementary Fig. 6 ). On the other hand, n -type conductive ultrananocrystalline diamond films prepared under hydrogen-poor conditions have achieved high electron mobility via oxygen ion doping [33] . The transport of electrons on a dimer surface is highly anisotropic, with the conductivity being much lower than that of our tube array surface, as implied by their band dispersions and calculated effective masses ( Supplementary Fig. 7 ; Supplementary Table 2 ). This indicates that the high n -type conductivity of ultrananocrystalline diamond films might be due to the formation of a TA1 surface structure. This was tested by an investigation of the formation mechanism of the TA1 surface under hydrogen-poor conditions on top of an initial dimer surface ( Supplementary Fig. 8 ). The adsorption of C 2 molecules [34] onto the dimer surface can lead to the formation of TA1 without any obvious transition barrier, while the continuous growth of the dimer structure would require a large energy barrier of 2–3 eV to be overcome [35] . This calculation proposes a viable synthesis route of the TA1 surface structure. Our finding of a previously unknown formation of self-assembled CNTs on the diamond (100) surface highlights the power of the intelligent surface structure-searching method developed here and reveals the chemical complexity of a seemingly simple system. Such methods would allow unusual surface chemistry to be explored unbiased by any chemical intuition, as demonstrated by the prediction of the longest known C–C σ bond in the self-assembled CNTs. Their intriguing transport properties, which feature different dimensionality for electron and hole carriers, and their potential applications in novel electronics urge the experimental exploration of these self-assembled CNTs under various controllable conditions. We show that the surface itself can be very important in nanoelectronics as it can become a functional part of a device. DFT calculations The supercell method was used to calculate surface energy, where the surface is represented by a finite-length slab. Both hydrogen passivation and symmetric slabs are used and they produce similar results. Each slab is separated from its neighbouring slabs in the (001) direction by at least 25 Å of vacuum and the slab contains 12 and 18 monolayers of C atoms for hydrogen passivation and symmetric models, respectively. Surface reconstruction structure searching was performed with various surface supercells of 2 × 1, 2 × 2, 3 × 1, 3 × 2, 3 × 3 and 4 × 4. Structure relaxations, electronic band structure, DOS and ELF calculations were performed within the framework of DFT as implemented by VASP (Vienna Ab initio Simulation Package) code [36] . Г-centred scheme was used for the Brillouin zone integration, and we used 4 × 4 × 1 K-point mesh. The cutoff energy for the expansion of wavefunction into plane waves was set to 900 eV for static total energy calculations, and for reducing computational cost, we adopt the cutoff energy of 600 eV for phonon calculations. Generalized gradient approximation with the PBE functional [24] and projector augmented wave potentials [37] was adopted to further relax the previously found surface structures. HSE hybrid functional [28] was used to calculate the band structures and total energies of selected structures. Besides the well-accepted PBE functional, many other functionals have also been used to confirm our result, and all of which give similar trend ( Supplementary Table 1 ). We also calculated the vibrational modes of CNTs and dimer surface structures within the quasi-harmonic approximation and evaluated the corresponding contributions to the free energies. As illustrated in Supplementary Fig. 11 , choices of cutoff energy for plane wave expansions, vacuum region between two neighbouring slabs, and the number of atomic layers per slab gave rise to the well-converged total energies at few meV per (1 × 1) unit cell. Electron-counting rule ECR has been used as an effective guide in conceiving the surface structures of insulator and semiconductors. It states that the number of electrons at the surface should be such that all surface bonding states and all anion DB states are occupied and that all cation DB states are empty. For surfaces of semiconductor with a sizable gap, anion DB states usually occur low in the gap, while cation DB states high in the gap. We developed a formula of ECR that explicitly display the alien atoms and bonds at the surface. By implementing this ECR formula, we greatly improved the efficiency of structure search. To clearly illustrate this general formula of ECR, we take the surface of an arbitrary binary compound A m B n as an example. In the chemical formula of A m B n , A denotes cation atom and B anion atom with valence-state + n and − m , respectively. We assume the surface also absorbs one kind of alien atom D with s valence electrons, and it is anion like. Taking an ideal surface of A m B n as the reference surface, the number of electrons from the surface and from the deposited atoms can be counted as: in which, N A , N B and N D are the number of A , B and D atoms on the reference surface, and is the number of electrons provided by the reference surface. One may notice that the choice of reference surface is not unique. However, as we will show later, it will not affect the result. The surface electrons can be counted from the number of DBs, for example, for A – B single bonds, each A atom will provide 2 n /( n +8− m ) electrons, while each B atom will provide 2(8− m )/( n +8− m ). Next, we count the number of electrons needed to fill all bonding states and anion DB states: in which N B ,DB and N D ,DB are the number of DB states of B atoms and deposited anion D atoms, respectively. N A – B , N D – A and N A – A are the number of A – B , D – A and A – A bonds. We can eliminate N B ,DB and N D ,DB according to the fact that anions need to be surrounded by an octet of electrons, that is, The number of excess electrons δ = n e – n b that are left after all bonding states and anion DB states are filled is then given by Following the same procedure, we can also obtain a similar formula for cation deposited atoms, the excess electrons are: These formulas show that contributions from different species cancel out if atoms satisfy stoichiometry (see the second item ofequations (5) and (6)). It is obvious that each part inequations (5) and (6) is linearly combined, so we could expand this rule to elemental solid and compounds with arbitrary stoichiometry: The summation in the second term is over all species of atoms deposited on the surface, N i denotes the number of the i th kind atom; v i is its atomic valence. The third term is summation over all kind of singular bonds; M j stands for the number of the j th kind of bonds, Δ j equals −1 for anion–anion bonds or 1 cation–cation bonds. How to cite this article: Lu, S. et al. Self-assembled ultrathin nanotubes on diamond (100) surface. Nat. Commun. 5:3666 doi: 10.1038/ncomms4666 (2014).